Total synthesis of mycobacterial arabinogalactan containing 92 monosaccharide units Carbohydrates are diverse bio-macromolecules with highly complex structures that are involved in numerous biological processes. Well-defined carbohydrates obtained by chemical synthesis are essential to the understanding of their functions. However, synthesis of carbohydrates is greatly hampered by its insufficient efficiency. So far, assembly of long carbohydrate chains remains one of the most challenging tasks for synthetic chemists. Here we describe a highly efficient assembly of a 92-mer polysaccharide by the preactivation-based one-pot glycosylation protocol. Several linear and branched oligosaccharide/polysaccharide fragments ranging from 5-mer to 31-mer in length have been rapidly constructed in one-pot manner, which enables the first total synthesis of a biologically important mycobacterial arabinogalactan through a highly convergent [31+31+30] coupling reaction. Our results show that the preactivation-based one-pot glycosylation protocol may provide access to the construction of long and complicated carbohydrate chains. Carbohydrates are involved in many key biological processes, such as cell signaling, cell proliferation and differentiation and viral and bacterial infections, as well as immunoresponse [1] , [2] , [3] . Naturally occurring carbohydrates and glycoconjugates usually exist in microheterogeneous forms, making the isolation of pure carbohydrates and glycoconjugates from natural sources difficult or even impossible in most cases. Therefore, chemical synthesis becomes the main approach to obtain well-defined carbohydrates [4] , [5] , [6] , [7] . However, unlike peptides and oligonucleotides, which can be routinely prepared by automated solid-phase synthesizers, the oligosaccharide synthesis is much more difficult. The major challenge for oligosaccharide preparation is the regio- and stereochemistry [8] , [9] issues in each glycosidic bond formation, making oligosaccharide synthesis a tedious and time-consuming process. Therefore, oligosaccharide synthesis becomes a daunting task, especially when polysaccharides are chosen as the target molecules. Indeed, only a few examples of the synthesis of oligosaccharide sequences containing >20 units have been reported over the past few decades [10] , [11] , [12] , [13] , [14] , [15] , [16] , [17] , [18] . These syntheses are challenging because multiple steps of protective group manipulation and intermediate purification are required in most cases. Arabinogalactan is an essential structural constituent of mycobacterial cell wall, which plays critical roles in the infectivity and pathogenicity of Mycobacterium tuberculosis [19] . Based on experiments and analyses [20] , [21] , [22] , the primary structure of arabinogalactan has been established as a linear galactan composed of about 30 alternating β -(1→5)-linked and β -(1→6)-linked D -galactofuranose (Gal f ) residues, to which up to two [22] highly branched arabinan chains (each containing 31 D -arabinofuranose (Ara f ) residues) are attached. The arabinogalactan motifs are useful probes for investigating the biosynthesis of mycobacterial cell wall, especially for characterization of the enzymes that process this polysaccharide, and those enzymes are attractive targets for the development of new antituberculosis drugs [23] . To this end, some solution phase [14] , [15] , [24] , [25] , [26] , [27] and automated solid-phase [28] strategies have been developed for the assembly of motifs up to 22 residues, among which the Lowary group [14] and Ito group [15] have elegantly synthesized the docosasaccharide arabinan motif via the convergent [5+5+12] and [7+7+8] coupling strategies, respectively. While almost all these syntheses relied upon the stepwise synthesis of oligosaccharide fragments, the object of this study is to achieve the total synthesis of the whole complex polysaccharide rather than the truncated fragments in an efficient way. In the preactivation-based one-pot glycosylation strategy, several glycosyl donors are allowed to react sequentially in the same vessel regardless of the anomeric reactivities, generating a single oligosaccharide as the main product, which can significantly simplify the synthetic process and increase the overall efficiency [29] . Herein, by utilizing the preactivation-based one-pot glycosylation protocol, we report the first total synthesis of a biologically important mycobacterial arabinogalactan composed of 92 monosaccharide units. Our synthetic strategy involves: (1) several scalable one-pot coupling reactions to generate the linear and branched oligosaccharide fragments, (2) the stereoselective β -arabinofuranosylation by preactivation protocol, (3) the further one-pot coupling reactions of oligosaccharide fragments for the rapid assembly of polysaccharides up to 31-mer, and (4) the convergent [31+31+30] coupling reaction for the final construction of the target polysaccharide. Retrosynthetic analysis The target polysaccharide arabinogalactan 1 was disconnected into two sizeable fragments, that is, the linear Gal f 30 acceptor 2 and the branched Ara f 31 donor 3 ( Fig. 1 ). It was conceived that Gal f 30 acceptor 2 would be rapidly assembled via a five-component one-pot coupling of several oligosaccharide fragments 4 – 7 . As for the synthesis of Ara f 31 donor 3 , oligosaccharide fragments 10 – 12 were designed to carry out a four-component one-pot glycosylation reaction. For the preparation of heptasaccharide 10 , thioglycoside donors 13a – c and thioglycoside acceptor 14 were planned for the construction of the challenging β -arabinofuranosyl linkages. Finally, it was expected that all the oligosaccharide fragments ( 8 , 9 , 15 – 17 ) would be accessible by the preactivation-based one-pot oligosaccharide synthesis starting from various monosaccharide building blocks. Overall, it was anticipated that the major challenge of our plan towards the total synthesis of arabinogalactan 1 would rely on the efficiency of one-pot glycosylation reactions, especially when large oligosaccharide fragments were attempted as the components in one-pot coupling reactions. 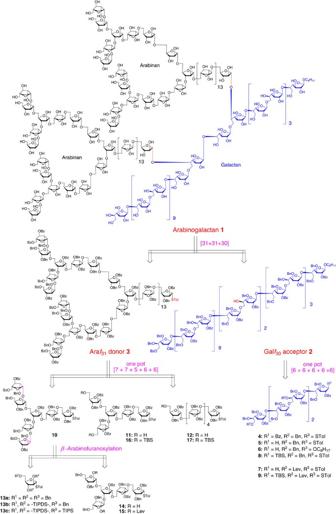Figure 1: The structure of mycobacterial arabinogalactan 1 and its retrosynthetic analysis. Bn, benzyl; Bz, benzoyl; Lev, levulinoyl; TBS,tert-butyldimethylsilyl; TIPDS, tetraisopropyldisiloxanylidene; TIPS, triisopropylsilyl; Tol,p-tolyl. Figure 1: The structure of mycobacterial arabinogalactan 1 and its retrosynthetic analysis. Bn, benzyl; Bz, benzoyl; Lev, levulinoyl; TBS, tert -butyldimethylsilyl; TIPDS, tetraisopropyldisiloxanylidene; TIPS, triisopropylsilyl; Tol, p -tolyl. Full size image Synthesis of Gal f 30 acceptor 2 To test our one-pot strategy for oligosaccharide synthesis, three monosaccharide building blocks 18 – 20 were designed and synthesized ( Supplementary Fig. 1 ). Using these building blocks, the assembly of hexasaccharide 8 in a six-component one-pot manner ( 18 + 19 + 20 + 19 + 20 + 19 ) by preactivation protocol was tried, which should be rather challenging as up to five glycosidic linkages must be correctly constructed. To our delight, when promoted by stoichiometric p -toluenesulfenyl chloride/silver triflate ( p -TolSCl/AgOTf) [29] , all glycosylation steps underwent smoothly and none of the side products interfered with the reaction. After optimization of the reaction conditions, hexasaccharide 8 was obtained in 63% overall yield and on a perfect scale (1.07 g) within several hours ( Fig. 2a ). The desilylation of 8 provided 5 (85% yield), which was re-protected with benzoyl group to give 4 in 96% yield. Subsequently, the coupling reaction of 8 with 1-octanol afforded 21 (91% yield), which was followed by desilylation to provide 6 in 87% yield. 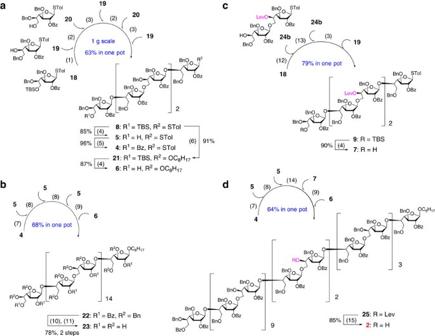Figure 2: Synthesis of Galf30acceptor 2. (a) Synthesis of oligosaccharides4–6; (b) Synthesis of 30-mer galactan23; (c) Synthesis of hexasaccharide7; (d) Synthesis of Galf30acceptor2. Reagents and conditions: (1) TTBP, 4 Å MS, CH2Cl2,p-TolSCl, AgOTf, then19, −78 °C to room temperature; (2)p-TolSCl, AgOTf, then20, −78 °C to room temperature; (3)p-TolSCl, AgOTf, then19, −78 °C to room temperature; (4) HF-pyridine, THF/H2O (10:1), 35 °C; (5) Bz2O, DMAP, pyridine, CH2Cl2, reflux; (6)p-TolSCl, AgOTf, TTBP, 1-octanol, 4 Å MS, CH2Cl2, −78 °C; (7) TTBP, 4 Å MS, CH2Cl2,p-TolSCl, AgOTf, then5, −78 °C to room temperature; (8)p-TolSCl, AgOTf, then5, −78 °C to room temperature; (9)p-TolSCl, AgOTf, then6, −78 °C to room temperature; (10) NaOCH3, CH3OH/CH2Cl2(2:1); (11) Pd/C, H2, EtOAc/THF/1-PrOH/H2O (2:1:1:1); (12) TTBP, 4 Å MS, CH2Cl2,p-TolSCl, AgOTf, then24b, −78 °C to room temperature; (13)p-TolSCl, AgOTf, then24b, −78 °C to room temperature; (14)p-TolSCl, AgOTf, then7, −78 °C to room temperature; (15) H2NNH2-AcOH, THF/CH3OH (10:1). DMAP, 4,4-dimethylaminopyridine; MS, molecular sieves; TTBP, 2,4,6-tri-tert-butylpyrimidine. Figure 2: Synthesis of Gal f 30 acceptor 2. ( a ) Synthesis of oligosaccharides 4 – 6 ; ( b ) Synthesis of 30-mer galactan 23 ; ( c ) Synthesis of hexasaccharide 7 ; ( d ) Synthesis of Gal f 30 acceptor 2 . Reagents and conditions: (1) TTBP, 4 Å MS, CH 2 Cl 2 , p -TolSCl, AgOTf, then 19 , −78 °C to room temperature; (2) p -TolSCl, AgOTf, then 20 , −78 °C to room temperature; (3) p -TolSCl, AgOTf, then 19 , −78 °C to room temperature; (4) HF-pyridine, THF/H 2 O (10:1), 35 °C; (5) Bz 2 O, DMAP, pyridine, CH 2 Cl 2 , reflux; (6) p -TolSCl, AgOTf, TTBP, 1-octanol, 4 Å MS, CH 2 Cl 2 , −78 °C; (7) TTBP, 4 Å MS, CH 2 Cl 2 , p -TolSCl, AgOTf, then 5 , −78 °C to room temperature; (8) p -TolSCl, AgOTf, then 5 , −78 °C to room temperature; (9) p -TolSCl, AgOTf, then 6 , −78 °C to room temperature; (10) NaOCH 3 , CH 3 OH/CH 2 Cl 2 (2:1); (11) Pd/C, H 2 , EtOAc/THF/1-PrOH/H 2 O (2:1:1:1); (12) TTBP, 4 Å MS, CH 2 Cl 2 , p -TolSCl, AgOTf, then 24b , −78 °C to room temperature; (13) p -TolSCl, AgOTf, then 24b , −78 °C to room temperature; (14) p -TolSCl, AgOTf, then 7 , −78 °C to room temperature; (15) H 2 NNH 2 -AcOH, THF/CH 3 OH (10:1). DMAP, 4,4-dimethylaminopyridine; MS, molecular sieves; TTBP, 2,4,6-tri- tert -butylpyrimidine. Full size image With hexasaccharides 4 – 6 in hand, the further iterative one-pot glycosylation was performed. The five-component one-pot coupling of these oligosaccharides ( 4 + 5 + 5 + 5 + 6 ) was realized successfully, producing the 30-mer polysaccharide 22 in 68% overall yield ( Fig. 2b ). It was noteworthy that some deletion sequences were difficult to be removed by column chromatography on silica gel. Gratifyingly, given the difference in molecular weight between the deletion sequences and desired product, size exclusion chromatography was then used to obtain the pure 30-mer polysaccharide 22 ( Supplementary Fig. 2 ). The identity of 22 was confirmed by its nuclear magnetic resonance (NMR) and matrix-assisted laser desorption/ionization–time of flight (MALDI-TOF) mass spectra (see Supplementary Information for details). Finally, the global deprotection of 22 via successive debenzoylation and debenzylation provided the 30-mer galactan 23 ([M+Na] + m / z calcd. for 5017.4, found: 5018.1). Having established a highly efficient one-pot approach to the synthesis of polysaccharide up to 30-mer, we turned to accomplish the construction of Gal f 30 acceptor 2 . As shown in Fig. 1 , an additional hexasaccharide 9 equipped with two levulinoyl groups was needed. Initially, monosaccharide 24a ( Supplementary Fig. 3 ) was designed as a building block for a six-component one-pot assembly of 9 . However, the efforts failed due to the migration of levulinoyl group from the O -5 to O -6 position. As an alternative route, disaccharide 24b was synthesized ( Supplementary Fig. 3 ). Therefore, a four-component one-pot coupling reaction ( 18 + 24b + 24b + 19 ) finally gave the desired hexasaccharide 9 in 79% yield ( Fig. 2c ), which was subjected to desilylation to afford 7 (90% yield). Subsequently, polysaccharide 25 was assembled in a five-component one-pot manner as described in the construction of 22 by coupling the oligosaccharide fragments ( 4 + 5 + 5 + 7 + 6 ) in 64% overall yield ( Fig. 2d ). Exposure of 25 to hydrazine acetate successfully fulfilled the preparation of the desired Gal f 30 acceptor 2 (85% yield). Synthesis of Ara f 31 donor 3 The assembly of the branched Ara f 31 donor 3 required three oligosaccharide intermediates, that is, β -Ara f -containing heptasaccharide 10 , branched pentasaccharide 11 and linear hexasaccharide 12 . For this purpose, a set of arabinofuranosyl building blocks ( 13a – c , 26 – 29 ) were designed and synthesized ( Supplementary Fig. 4 ). A six-component iterative one-pot glycosylation of monosaccharides 26 and 27 ( 26 + 27 + 27 + 27 + 27 + 27 ) afforded hexasaccharide 17 in excellent yield (73%) and on gram scale (1.20 g) ( Fig. 3a ). The desilylation of 17 resulted in the desired hexasaccharide 12 (92% yield). Likewise, the one-pot coupling reaction of building blocks 26 , 28 (ref. 30 ) and 27 provided a branched pentasaccharide 16 very smoothly (78% yield), which was further converted into diol 11 by desilylation in 95% yield ( Fig. 3b ). For the preparation of heptasaccharide 10 , another diol 14 was required. Initially, the glycosyl donor 29a (ref. 31 ) with chloroacetyl group at the O -2 position was chosen for the one-pot construction of pentasaccharide 15a ( Supplementary Table 1 ), but the overall yield was moderate (43%). Fortunately, when the donor 29 equipped with a levulinoyl group was employed for the one-pot glycosylation reaction, pentasaccharide 15 was rapidly assembled in 76% overall yield ( Fig. 3b ). Ultimately, deacylation of 15 gave diol 14 (94% yield). 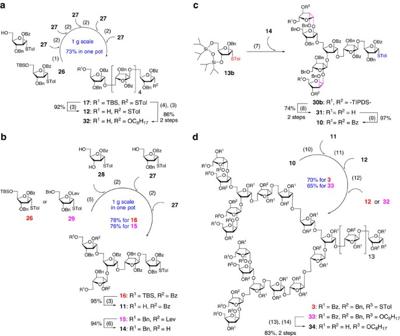Figure 3: Synthesis of Araf31donor 3. (a) Synthesis of oligosaccharides12and32; (b) Synthesis of diols11and14; (c) Synthesis of heptasaccharide10; (d) Synthesis of Araf31donor3and 31-mer arabinan34. Reagents and conditions: (1) TTBP, 4 Å MS, CH2Cl2,p-TolSCl, AgOTf, then27, −78 °C to room temperature; (2)p-TolSCl, AgOTf, then27, −78 °C to room temperature; (3) TBAF, AcOH, THF; (4)p-TolSCl, AgOTf, TTBP, 1-octanol, 4 Å MS, CH2Cl2, −78 °C; (5) TTBP, 4 Å MS, CH2Cl2,p-TolSCl, AgOTf, then28, −78 °C to room temperature; (6) H2NNH2-AcOH, THF/CH3OH (10:1); (7)p-TolSCl, AgOTf, then14, −78 °C; (8) TBAF, THF; (9) Bz2O, DMAP, pyridine, CH2Cl2, reflux; (10) TTBP, 4 Å MS, CH2Cl2,p-TolSCl, AgOTf, then11, −78 °C to room temperature; (11)p-TolSCl, AgOTf, then12, −78 °C to room temperature; (12)p-TolSCl, AgOTf, then12or32, −78 °C to room temperature; (13) NaOCH3, CH3OH/CH2Cl2(2:1); (14) Pd/C, H2, EtOAc/THF/1-PrOH/H2O (2:1:1:1). TBAF, tetra-n-butylammonium fluoride. Figure 3: Synthesis of Ara f 31 donor 3. ( a ) Synthesis of oligosaccharides 12 and 32 ; ( b ) Synthesis of diols 11 and 14 ; ( c ) Synthesis of heptasaccharide 10 ; ( d ) Synthesis of Ara f 31 donor 3 and 31-mer arabinan 34 . Reagents and conditions: (1) TTBP, 4 Å MS, CH 2 Cl 2 , p -TolSCl, AgOTf, then 27 , −78 °C to room temperature; (2) p -TolSCl, AgOTf, then 27 , −78 °C to room temperature; (3) TBAF, AcOH, THF; (4) p -TolSCl, AgOTf, TTBP, 1-octanol, 4 Å MS, CH 2 Cl 2 , −78 °C; (5) TTBP, 4 Å MS, CH 2 Cl 2 , p -TolSCl, AgOTf, then 28 , −78 °C to room temperature; (6) H 2 NNH 2 -AcOH, THF/CH 3 OH (10:1); (7) p -TolSCl, AgOTf, then 14 , −78 °C; (8) TBAF, THF; (9) Bz 2 O, DMAP, pyridine, CH 2 Cl 2 , reflux; (10) TTBP, 4 Å MS, CH 2 Cl 2 , p -TolSCl, AgOTf, then 11 , −78 °C to room temperature; (11) p -TolSCl, AgOTf, then 12 , −78 °C to room temperature; (12) p -TolSCl, AgOTf, then 12 or 32 , −78 °C to room temperature; (13) NaOCH 3 , CH 3 OH/CH 2 Cl 2 (2:1); (14) Pd/C, H 2 , EtOAc/THF/1-PrOH/H 2 O (2:1:1:1). TBAF, tetra- n -butylammonium fluoride. Full size image Our attention was then turned to the synthesis of heptasaccharide 10 , which involved the stereocontrolled installation of two challenging β -arabinofuranosyl linkages. Among a number of innovative glycosyl donors developed by several groups [25] , [31] , [32] , [33] , [34] , [35] , [36] , [37] , perbenzyl-protected thioglycoside 13a (ref. 25 ) and 3,5- O -tetraisopropyldisiloxanylidene-protected thioglycosides 13b , c (ref. 31 ) were synthesized for the current purpose ( Supplementary Table 2 ). Although these donors proved useful for direct β -arabinofuranosylation, whether they could be subjected to thioglycoside acceptor 14 under the donor-preactivation conditions [38] remained to be explored. After some optimization, the best result arised when 4.0 equiv. of 13b was preactivated by p -TolSCl/AgOTf and subsequently glycosylated with 1.0 equiv. of diol 14 , delivering heptasaccharide 30b with good stereoselectivity ( β,β -isomer/other isomers=9/1). Removal of the silyl groups in 30b afforded 31 (74% over two steps, Fig. 3c ), in which the newly formed β -arabinofuranosyl linkages were confirmed by the 13 C NMR spectrum (appearance at 99.6 and 99.1 p.p.m.) [39] . Finally, the re-protection of 31 with benzoyl groups yielded the desired heptasaccharide 10 (97% yield). With oligosaccharide building blocks 10 – 12 in hand, the assembly of Ara f 31 donor 3 by preactivation-based one-pot glycosylation protocol was attempted. This one-pot reaction was expected to be more challenging due to the steric hindrance in the double glycosylation of Ara f 5 acceptor 11 using Ara f 7 donor 10 . Surprisingly, the reaction proceeded smoothly when 2.3 equiv. of 10 was reacted with 1.0 equiv. of 11 , delivering an Ara f 19 intermediate, which was sequentially coupled with two Ara f 6 acceptors 12 in a single flask without any intermediate isolation to afford the Ara f 31 donor 3 in 70% overall yield ( Fig. 3d ). To further confirm the identity of this 31-mer polysaccharide, an Ara f 6 acceptor 32 bearing an alkyl group at the reducing end was synthesized ( Fig. 3a ). Thus a four-component one-pot coupling reaction of oligosaccharides 10 – 12 and 32 gave a similar 31-mer polysaccharide 33 in 65% yield ( Fig. 3d ), which was fully deprotected via deacylation and hydrogenolysis to afford the arabinan 34 ([M+Na] + monoisotopic m / z calcd. for 4246.4, found: 4246.3; [M+K] + monoisotopic m / z calcd. for 4262.4, found: 4262.2). Gratifyingly, the 1 H and 13 C NMR data of 34 were found to be identical with previous reports [14] , [40] except for the differences in some repeating units. Assembly of arabinogalactan 1 Our final task was the glycosylation of Gal f 30 acceptor 2 with Ara f 31 donor 3 to finish the assembly of target polysaccharide. To the best of our knowledge, no glycosylation reactions between polysaccharide sequences composed of >20 units were reported to date. For the planned [31+31+30] coupling reaction, it was anticipated that the biggest challenge would come from the steric hindrance by the bulky size of both the donor and acceptor, especially when a double glycosylation was required. Indeed, when a wide variety of promoter systems such as p -TolSCl/AgOTf [29] , NIS/AgOTf [41] , NIS/TfOH [42] , N -( p -methylphenylthio)-ɛ-caprolactam/Tf 2 O [43] , TBPA [44] , Ph 3 Bi(OTf) 2 (ref. 45 ), BSP/Tf 2 O [46] and Ph 2 SO/Tf 2 O [47] were examined ( Supplementary Table 3 ), no double glycosylation product or only some monoglycosylation product was observed before the donor decomposed, prompting us to further screen the reaction conditions. Encouragingly, it was found that benzenesulfinyl morpholine/triflic anhydride (BSM/Tf 2 O) [48] developed by our group is the most effective promoter. And indeed, when promoted by BSM/Tf 2 O, this double glycosylation was extremely clean and complete (indicated by thin-layer chromatography analysis), delivering the fully protected arabinogalactan 35 in 84% yield ( Fig. 4 ). Although signals of the anomeric protons in 1 H NMR spectrum were obscured due to the extensive overlapping, the anomeric carbons were distinctive in 13 C NMR spectrum (all anomeric carbons of α -Ara f residues and β -Gal f residues were between 105 and 107 p.p.m., and anomeric carbons of β -Ara f residues appeared at 101.0 and 100.6 p.p.m.). The identity of 35 was further supported by its MALDI-TOF mass spectrum ([M+Na] + m / z calcd. for 33885.4, found: 33884.7). Finally, the global deprotection of 35 by the successive deacylation and hydrogenolysis was conducted, affording the target polysaccharide arabinogalactan 1 successfully. 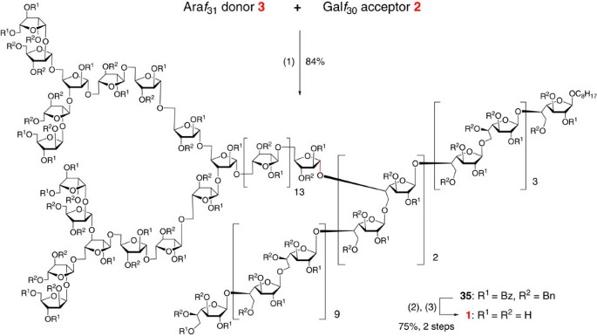Figure 4: Assembly of arabinogalactan 1. Reagents and conditions: (1) BSM, Tf2O, 4 Å MS, CH2Cl2, −40 °C; (2) NaOCH3, CH3OH/THF (2:1); (3) Pd/C, H2, EtOAc/THF/1-PrOH/H2O (2:1:1:1). BSM, benzenesulfinyl morpholine. Figure 4: Assembly of arabinogalactan 1. Reagents and conditions: (1) BSM, Tf 2 O, 4 Å MS, CH 2 Cl 2 , −40 °C; (2) NaOCH 3 , CH 3 OH/THF (2:1); (3) Pd/C, H 2 , EtOAc/THF/1-PrOH/H 2 O (2:1:1:1). BSM, benzenesulfinyl morpholine. Full size image We have developed a concise and highly efficient strategy for the first total synthesis of 92-mer mycobacterial arabinogalactan 1 . This work not only represents the longest well-defined carbohydrate chain synthesis up to date, but also provides useful compounds as probes for further investigations on mycobacterial cell wall-related biological events. Our synthetic strategy highlights a series of efficient preactivation-based one-pot glycosylation reactions to minimize the synthetic steps, the stereoselective β -arabinofuranosylation by preactivation protocol and the convergent [31+31+30] double glycosylation reaction, thus offering a straightforward access to the target polysaccharide. Our work may open an avenue to the synthesis of complex polysaccharides with biological importance that are either difficult or impossible to access through isolation or semisynthesis. General The complete experimental details and compound characterization data can be found in Supplementary Methods . For the NMR, HPLC and MALDI-TOF mass spectra of the compounds in this article, see Supplementary Figs 5–126 . General procedure for preactivation-based one-pot glycosylation reaction A mixture of glycosyl donor, TTBP and freshly activated 4 Å molecular sieves in anhydrous CH 2 Cl 2 under argon atmosphere was stirred for 20 min at room temperature and cooled to −78 °C. After 5 min, stoichiometric amount of p -TolSCl was added to the mixture, followed by the addition of AgOTf. After another 5 min, a solution of glycosyl acceptor in anhydrous CH 2 Cl 2 was slowly added. The resulting mixture was slowly warmed to room temperature within 2 h, stirred for another 20 min and cooled back to −78 °C. The glycosylation operation mentioned above was repeated until the generation of the desired product. Data availability The authors declare that the data supporting the findings of this study are available within the article and its Supplementary Information files. And all data are available from the authors upon reasonable request. How to cite this article: Wu, Y. et al . Total synthesis of mycobacterial arabinogalactan containing 92 monosaccharide units. Nat. Commun. 8, 14851 doi: 10.1038/ncomms14851 (2017). Publisher’s note : Springer Nature remains neutral with regard to jurisdictional claims in published maps and institutional affiliations.